G-quadruplex structures are stable and detectable in human genomic DNA The G-quadruplex is an alternative DNA structural motif that is considered to be functionally important in the mammalian genome for transcriptional regulation, DNA replication and genome stability, but the nature and distribution of G-quadruplexes across the genome remains elusive. Here, we address the hypothesis that G-quadruplex structures exist within double-stranded genomic DNA and can be explicitly identified using a G-quadruplex-specific probe. An engineered antibody is employed to enrich for DNA containing G-quadruplex structures, followed by deep sequencing to detect and map G-quadruplexes at high resolution in genomic DNA from human breast adenocarcinoma cells. Our high sensitivity structure-based pull-down strategy enables the isolation of genomic DNA fragments bearing single, as well as multiple G-quadruplex structures. Stable G-quadruplex structures are found in sub-telomeres, gene bodies and gene regulatory regions. For a sample of identified target genes, we show that G-quadruplex-stabilizing ligands can modulate transcription. These results confirm the existence of G-quadruplex structures and their persistence in human genomic DNA. Guanine-rich DNA can form four-stranded DNA structures called G-quadruplexes [1] . Genome-wide bioinformatics analyses show that G-quadruplex sequence motifs are prevalent in the human genome and are enriched in gene regulatory regions and gene bodies, and in repetitive sequences, such as telomeres [2] , [3] , [4] , [5] . Such studies have sparked the need to map folded G-quadruplex structures carried by the genome in an explicit way. A number of studies have linked G-quadruplexes to key biological processes such as transcriptional regulation, DNA replication and genome stability, leading to their exploration as therapeutic targets [6] , [7] . G-quadruplexes are stable under near-physiological conditions in vitro , and a central challenge in the field has been to establish whether such structures can form in genomic DNA. Support for G-quadruplex formation has emerged from the use of small molecule G-quadruplex-targeting ligands to perturb cellular function [8] . Such small molecules have been shown to localize at telomeres [9] and have been used to enrich for human telomeric DNA [10] . Engineered proteins, including the hf2 single-chain antibody [11] and the Gq1 zinc finger protein [12] have been generated as molecular probes that are exquisitely G-quadruplex-structure specific. Indeed, a G-quadruplex antibody was previously employed to visualize G-quadruplex formation at the millions of telomeres present in the macronuclei of ciliates [13] and in human cells [14] . Here, we sought to explicitly demonstrate that G-quadruplex structures exist within double-stranded genomic DNA using a G-quadruplex-specific probe. We report the presence and localization of stable G-quadruplex structures in genomic DNA isolated from human cells. The hf2 antibody pulls down DNA G-quadruplex structures We employed a G-quadruplex-specific antibody to enrich for genomic DNA fragments containing folded G-quadruplex structures, followed by deep sequencing of the isolated DNA to identify the regions comprising G-quadruplex structures. We used the single-chain antibody, hf2, which we previously showed binds to a range of folded DNA G-quadruplex structures formed by synthetic oligonucleotides, but with negligible binding to single- and double-stranded DNA [11] . After re-affirming the binding specificity of hf2 by ELISA ( Supplementary Fig. S1 ), we confirmed that in solution hf2 could pull-down DNA G-quadruplex structures formed by synthetic DNA oligonucleotides ( Supplementary Figs S2 and S3 ). The specificity of hf2 to enrich G-quadruplex structures was then confirmed using mixtures of G-quadruplex and non-G-quadruplex single-stranded or double-stranded DNA oligonucleotides. The gel shown in Fig. 1a ( Supplementary Fig. S3 ) confirms the specific capture of G-quadruplex-structured DNA (KIT-2) from such mixtures by hf2 without significant contaminating non-G-quadruplex DNA. We also showed that hf2 could specifically capture the telomeric G-quadruplex oligonucleotide, Htelo, in the presence of a 100-fold excess of double-stranded salmon sperm DNA ( Fig. 1a ), confirming the probe specificity and robust conditions for seeking such non-canonical structures from DNA of genomic complexity. 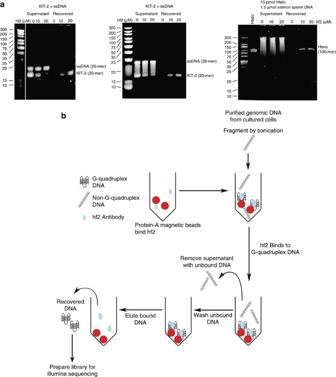Figure 1: The hf2 single-chain antibody specifically pulls down G-quadruplex oligonucleotides. (a) Pull-down of G-quadruplex oligonucleotides by hf2 analysed on TBE-urea gels. Left, KIT-2 G-quadruplex oligonucleotides but not single-stranded DNA are captured by hf2. Lane 1 shows the GeneRuler Ultra Low Range DNA Ladder (Thermo Scientific), lanes 2–4 show concentration-dependent depletion of KIT-2 quadruplex, but not single-stranded DNA (control) from the supernatant by hf2, lanes 5–7 show the specific recovery of KIT-2 quadruplex, but not single-stranded DNA with increasing hf2 concentration. Middle, KIT-2 G-quadruplex oligonucleotides but not double-stranded DNA are captured by hf2. Lane 1 shows the GeneRuler Ultra Low Range DNA Ladder, lanes 2–4 show concentration-dependent depletion of KIT-2 quadruplex, but not doubled-stranded DNA (control) from the supernatant by hf2, lanes 5–7 show the specific recovery of KIT-2 quadruplex, but not double-stranded DNA with increasing hf2 concentration. Right, Htelo G-quadruplex oligonucleotides are captured by hf2 in the presence of excess sonicated salmon sperm DNA. Lane 1 shows the Htelo oligonucleotide alone, lanes 2–4 show the unbound supernatant with different hf2 concentrations, lanes 5–7 show the specific recovery of KIT-2 quadruplex, but not double-stranded salmon sperm DNA. (b) Pull-down protocol used to isolate G-quadruplex DNA from genomic DNA with the hf2 antibody. Figure 1: The hf2 single-chain antibody specifically pulls down G-quadruplex oligonucleotides. ( a ) Pull-down of G-quadruplex oligonucleotides by hf2 analysed on TBE-urea gels. Left, KIT-2 G-quadruplex oligonucleotides but not single-stranded DNA are captured by hf2. Lane 1 shows the GeneRuler Ultra Low Range DNA Ladder (Thermo Scientific), lanes 2–4 show concentration-dependent depletion of KIT-2 quadruplex, but not single-stranded DNA (control) from the supernatant by hf2, lanes 5–7 show the specific recovery of KIT-2 quadruplex, but not single-stranded DNA with increasing hf2 concentration. Middle, KIT-2 G-quadruplex oligonucleotides but not double-stranded DNA are captured by hf2. Lane 1 shows the GeneRuler Ultra Low Range DNA Ladder, lanes 2–4 show concentration-dependent depletion of KIT-2 quadruplex, but not doubled-stranded DNA (control) from the supernatant by hf2, lanes 5–7 show the specific recovery of KIT-2 quadruplex, but not double-stranded DNA with increasing hf2 concentration. Right, Htelo G-quadruplex oligonucleotides are captured by hf2 in the presence of excess sonicated salmon sperm DNA. Lane 1 shows the Htelo oligonucleotide alone, lanes 2–4 show the unbound supernatant with different hf2 concentrations, lanes 5–7 show the specific recovery of KIT-2 quadruplex, but not double-stranded salmon sperm DNA. ( b ) Pull-down protocol used to isolate G-quadruplex DNA from genomic DNA with the hf2 antibody. Full size image Genome-wide pull-down of G-quadruplexes We then undertook to detect G-quadruplex structures in double-stranded genomic DNA isolated from human breast adenocarcinoma (MCF7) cells using the hf2 antibody as outlined schematically in Fig. 1b . If stable G-quadruplex structures exist within double-stranded genomic DNA, we reasoned that hf2 would selectively enrich such regions, leading to peaks in DNA sequencing that correspond to G-quadruplex motifs. The hf2 antibody probe was first immobilized onto protein-A Dynabeads then incubated with sonicated human genomic DNA, followed by elution of the captured DNA fragments and subsequent deep sequencing. Pull-down conditions were optimized by assessing telomere enrichment, as there is already substantial evidence for G-quadruplex structure formation at telomeres [13] , [15] . Selective qRT–PCR analysis of the repetitive telomeric sequences [16] compared with a region of the oestrogen receptor enhancer lacking predicted G-quadruplexes, showed that telomeric sequences were enriched by >20-fold in the pull-down DNA relative to control, providing proof-of-principle of the overall approach. Further controls confirmed that the buffer conditions used during genomic DNA isolation and sonication also do not induce or destroy G-quadruplex structures ( Supplementary Figs S4 and S5 ). The hf2-enriched genomic DNA library was then sequenced at high depth to identify DNA fragments containing a G-quadruplex structure. Sequencing reads from four independent libraries were aligned to the human genome and peaks called using the Model-based Analysis of ChIP-Seq (MACS) algorithm [17] . To identify enriched regions with high confidence and assess the reproducibility of the enrichment, we computed the quality metrics recently developed to assess ENCODE data [18] ( Supplementary Table S1 , Supplementary Fig. S6 ). The quality metrics of the G-quadruplex pull-down libraries were generally within the ENCODE acceptable thresholds, and are comparable to transcription factor ChIP-Seq data. Confirmation of G-quadruplex structures in identified peaks The sequence of the peaks across the genome was then examined for predicted G-quadruplex sequences by the G4-calculator algorithm [19] . The G4-calculator analyzes a fixed width sequence window for G-quadruplex-forming potential, defined as at least four runs of three or more guanines within 100 bases. The proportion of windows with G-quadruplex-forming potential is then computed for the entire length of the peak. The number of peaks with G-quadruplex-forming potential was significantly higher than expected by chance ( Supplementary Table S2 , Supplementary Figs S7 and S8 ). To identify consistently observed peaks, we considered only those in common between at least two of the four libraries. Of the enriched regions, the majority (568/768, 74.0%) had G-quadruplex-forming potential, and this compares favourably with the proportion of motif-containing peaks typically seen in ChIP-Seq for transcription factors, such as NRSF [20] . Although G4-calculator indicates which peaks have G-quadruplex-forming potential, it does not specify their precise position within the peak. To accurately map the genomic location of predicted G-quadruplexes within the peaks, we therefore used an alternative G-quadruplex prediction algorithm, quadparser [2] . Quadparser uses a more stringent consensus (G 3+ N 1–7 G 3+ N 1–7 G 3+ N 1–7 G 3+ ) by constraining loop lengths of the G-quadruplex to a maximum of seven bases. The number of peaks having a predicted G-quadruplex computed by quadparser was also found to be statistically significant ( Supplementary Table S3 , Supplementary Figs S9 and S10 ), giving 175 predicted G-quadruplex-containing peaks ( Fig. 2 , Supplementary Fig. S11 , Supplementary Table S4 ). 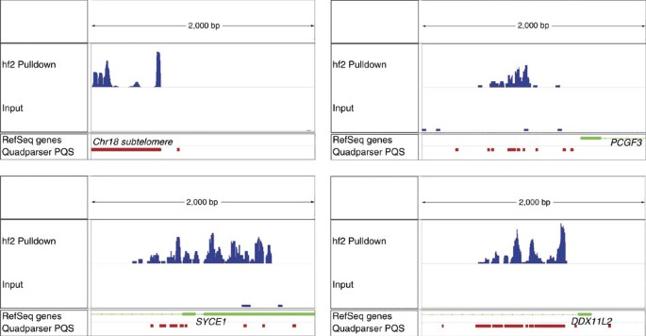Figure 2: Peaks identified by deep sequencing after pull-down with the anti-G-quadruplex hf2 antibody. Genome browser view of four peaks (blue) present compared with input and the overlap with G-quadruplex sequences predicted by quadparser (red). RefSeq gene is shown in green. The peaks map to different chromosomal locations including the sub-telomere (top left), gene promoter (top right), exon (bottom left) and intron (bottom right). Figure 2: Peaks identified by deep sequencing after pull-down with the anti-G-quadruplex hf2 antibody. Genome browser view of four peaks (blue) present compared with input and the overlap with G-quadruplex sequences predicted by quadparser (red). RefSeq gene is shown in green. The peaks map to different chromosomal locations including the sub-telomere (top left), gene promoter (top right), exon (bottom left) and intron (bottom right). Full size image As an independent evaluation of the binding specificity of hf2, we analysed the combined sequence reads from all libraries using the motif-finding algorithm, MEME [21] . This approach makes no a priori assumptions of the sequence types expected. Analysis of the top 200 peaks by enrichment over input showed that the most frequent MEME sequence motif calculated matches the G-quadruplex consensus ( Fig. 3a , Supplementary Fig. S12 ), and is thus consistent with the enrichment of potential G-quadruplex structures by our pull-down strategy. When MEME was used on the 200 most enriched peaks called in the input library or 200 random sequences from the genome, similar motifs were not observed ( Supplementary Fig. S12 ). As G-quadruplexes display characteristic circular dichroism (CD) spectroscopic signatures indicative of their structure [22] , we determined the structural characteristics of oligonucleotides with G-quadruplex-forming potential covering a set of pull-down peaks. Parallel G-quadruplexes display positive and negative peaks at 260 and 240 nm, respectively, while anti-parallel G-quadruplexes exhibit positive and negative peaks at 295 and 260 nm [23] . We analysed the CD spectra of a series of 44 non-overlapping oligonucleotides spanning all of the G-repeats, from two sub-telomeric peaks and two peaks elsewhere in the genome ( Supplementary Table S5 ). Forty-two showed CD spectra with a peak at 295 nm. These spectra are consistent with the majority of the sequences folding into either a hybrid-type G-quadruplex structure with mixed parallel/anti-parallel strands or a mixture of parallel and anti-parallel G-quadruplexes ( Fig. 3b , Supplementary Fig. S13 ). 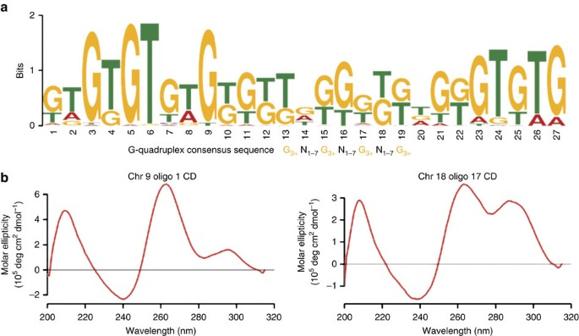Figure 3: Motif and CD analyses substantiate G-quadruplex identification. (a) Sequence logo of the most enriched motif as determined by MEME21(e-value=1.9e−190, expected value from MEME expectation maximization algorithm) found in the top 200 peaks ranked by enrichment (false discovery rate <0.05). The G-quadruplex consensus sequence is shown here for comparison. (b) Examples of CD spectra for two oligonucleotides from the identified peaks. Parallel G-quadruplexes display a characteristic peak at 263 nm and a trough at 240 nm, whereas anti-parallel G-quadruplexes show a peak at 295 nm. The CD spectra show characteristics of both parallel and anti-parallel G-quadruplexes indicative of hybrid-type G-quadruplexes or a mixture of parallel and anti-parallel G-quadruplexes. Figure 3: Motif and CD analyses substantiate G-quadruplex identification. ( a ) Sequence logo of the most enriched motif as determined by MEME [21] ( e -value=1.9e −190 , expected value from MEME expectation maximization algorithm) found in the top 200 peaks ranked by enrichment (false discovery rate <0.05). The G-quadruplex consensus sequence is shown here for comparison. ( b ) Examples of CD spectra for two oligonucleotides from the identified peaks. Parallel G-quadruplexes display a characteristic peak at 263 nm and a trough at 240 nm, whereas anti-parallel G-quadruplexes show a peak at 295 nm. The CD spectra show characteristics of both parallel and anti-parallel G-quadruplexes indicative of hybrid-type G-quadruplexes or a mixture of parallel and anti-parallel G-quadruplexes. Full size image Regulation of identified genes by a G-quadruplex ligand Having proven the presence of G-quadruplex structures in defined locations within genomic DNA, we next investigated the consequence of G-quadruplex formation at some of these explicit sites in cells. We selected an example set of eight genes ( ABCG1 , ACTN1 , DYSF , ELL , LRP1 , PVT1 , STARD8 and TOM1) , each with G-quadruplex structures, identified by hf2 enrichment, within 1 kb of the transcribed regions of the gene, in at least three libraries. G-quadruplex formation has been linked to the regulation of transcription and thus G-quadruplex stabilization by a ligand would be predicted to modulate transcription as has been exemplified in other studies [24] , [25] . We treated MCF7 cells with the highly specific G-quadruplex-stabilizing ligand, pyridostatin (PDS) [26] , and assessed changes in expression of the selected genes by qRT–PCR. Gene expression was normalized to the housekeeping gene RPLP0 , which contains no predicted G-quadruplexes and does not show a peak with hf2 pull-down. Nested analysis of variance showed PDS treatment caused a significant change in the expression of the selected genes ( P =4.9 × 10 −10 ). Six of the G-quadruplex-containing genes analysed had statistically significant changes in gene expression ( P <0.05, Student’s t -test) caused by ligand treatment, the remaining two genes also showed downregulation ( P -value<0.09, Student’s t -test) ( Fig. 4 ), while two control genes, ACTB1 and B2M , that were not enriched by hf2, showed no changes in gene expression. 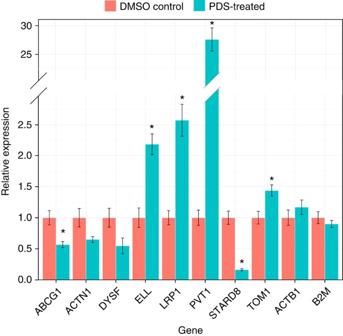Figure 4: Stabilizing small molecules modulate the expression of identified G-quadruplex-containing genes. qRT–PCR was used to examine the expression of selected genes, identified by hf2 pull-down to contain G-quadruplexes, in MCF7 cells that were treated in triplicate with the G-quadruplex-specific small molecule PDS or DMSO control. The mean and s.e. (error bars) of the relative expression levels of genes in PDS-treated and DMSO control are plotted on two different scales to show the different magnitudes of changes. Two genes in particular,PVT1andSTARD8, show large changes in gene expression in PDS-treated cells compared with controls. The Student’st-test was used to calculate statistical significance between PDS-treated and control cells. Asterisks indicate statistically significant changes in gene expression withP<0.05. TheP-values forABCG1, ACTN1, DYSF, ELL, LRP1, PVT1, STARD8, TOM1, ACTB1andB2Mare 0.0251, 0.0868, 0.0840, 0.0069, 0.0051, 0.0002, 0.0015, 0.0323, 0.3720 and 0.4189. Figure 4: Stabilizing small molecules modulate the expression of identified G-quadruplex-containing genes. qRT–PCR was used to examine the expression of selected genes, identified by hf2 pull-down to contain G-quadruplexes, in MCF7 cells that were treated in triplicate with the G-quadruplex-specific small molecule PDS or DMSO control. The mean and s.e. (error bars) of the relative expression levels of genes in PDS-treated and DMSO control are plotted on two different scales to show the different magnitudes of changes. Two genes in particular, PVT1 and STARD8 , show large changes in gene expression in PDS-treated cells compared with controls. The Student’s t -test was used to calculate statistical significance between PDS-treated and control cells. Asterisks indicate statistically significant changes in gene expression with P <0.05. The P -values for ABCG1, ACTN1, DYSF, ELL, LRP1, PVT1, STARD8, TOM1, ACTB1 and B2M are 0.0251, 0.0868, 0.0840, 0.0069, 0.0051, 0.0002, 0.0015, 0.0323, 0.3720 and 0.4189. Full size image The work presented here investigates the hypothesis that G-quadruplex structures are present and stable in human DNA. Using a structure-specific antibody, we have proven that G-quadruplex structures indeed persist in genomic DNA isolated from human cancer cells. Furthermore, we have mapped their locations in the genome at high resolution using deep sequencing. ChIP-Seq is a widely used method to map transcription factors and chromatin-associated protein binding sites in the genome, and metrics to assess data quality and analysis are becoming accepted [18] . Our G-quadruplex genomic DNA mapping approach has significant differences from the standard ChIP-Seq method for point-source peaks (for example, transcription factors). Therefore, we propose a workflow for G-quadruplex DNA sequencing experiment. First, before sequencing we recommend quantifying the telomere G-quadruplex enrichment by qRT–PCR, which should be preferably greater than 20-fold. Second, we suggest assessing the quality of G-quadruplex enriched libraries according to the ENCODE guidelines [18] as exemplified by Supplementary Table S1 . Third, a statistically significant proportion of the identified peaks should contain putative G-quadruplex sequences (as in Supplementary Figs S6 and S8 ). In the G-quadruplex mapping method, most peaks are only present in one library. This is due to the small number of bona fide peaks compared with the very large number of peaks that peak-calling algorithms generally produce, thus replicates are essential to identify consistently called peaks. We therefore recommend sequencing at least three independent biological replicates, and performing peak-calling with an established ChIP-Seq peak-caller, such as MACS. We suggest that only peaks below a P -value cutoff of 10 −5 (from MACS) and present in at least two libraries be used for further analyses. Computational methods have previously identified >370,000 individual sequence motifs in the human genome with the potential to form a G-quadruplex [2] . Such studies have raised the need to elucidate which of these potential structures actually form in the genome. Our work has definitively identified several genomic DNA regions that stably retain a folded G-quadruplex structure even after DNA isolation procedures. This particular study does not define an exhaustive list of all G-quadruplex structures that will form in the genome for a number of reasons. First, the hf2 antibody used in our experiments was selected against a particular G-quadruplex [11] , and although it does bind to several other G-quadruplex sequences, it is unlikely to recognize all G-quadruplex folds and sequences with equal affinity. Second, we hypothesize that the formation of some G-quadruplexes will be temporally coupled to functional processes, such as transcription and replication, thus structure formation may only be transient [14] . For example, helicases present in cells, such as PIF1, BLM, WRN and FANCJ, are known to resolve G-quadruplex structures at replication forks [27] , [28] , [29] , [30] and may be involved in controlling the lifetimes of such structure. Furthermore, the changing torsional stress in regions of the genome is also likely to have influence on the formation of such alternative structures during transcriptional events [31] , [32] . In our study, we have found examples of stable G-quadruplexes within 2 kb upstream of the transcriptional start site of several genes. This finding is in keeping with the predictions from bioinformatics studies that many of protein-coding genes may harbour a G-quadruplex in their upstream promoter regions [19] , [33] . Extensive biophysical and cellular experiments have previously lent support for G-quadruplex formation in the promoters of specific genes including KIT [34] , BCL2 [35] , VEGF [36] , MYC [37] and KRAS [38] . As we have provided evidence for the existence of stable G-quadruplexes in the promoter of a set of previously uninvestigated genes, these may prove to be valuable new targets for the exploration of G-quadruplex-mediated transcriptional regulation. Informatics analyses have also highlighted an enrichment of G-quadruplex-forming potential in 5′-UTRs, first introns and gene 3′ regions [5] , [39] . We have now furnished evidence for stable G-quadruplex formation within genes (219 genes). G-quadruplexes located within genes have previously been correlated with transcriptional pausing by RNA PolII [5] , and recently we have further demonstrated that small molecule targeting of G-quadruplexes leads to inhibition of SRC expression through transcriptional at pausing at G-quadruplexes positioned within the gene body [40] . Our current results have identified further G-quadruplexes present within other genes highlighting additional regions that may be important in transcriptional elongation. We also observed G-quadruplexes in the 3′ region of several genes (37 genes), a position where predicted G-quadruplexes have been previously associated with transcriptional termination through R-loop formation and resolution by the senataxin helicase [41] . The identification and localization of stable G-quadruplexes to gene regions of functional importance further reinforces the potentially wide role of G-quadruplex structures rather than G-rich sequences per se in regulating biological processes, such as transcriptional initiation, elongation and termination. We have now provided evidence of existence for an exemplary set of G-quadruplex structures identified by hf2 pull-down from genomic DNA. Furthermore, a sub-set of these genes containing a G-quadruplex were all shown to be susceptible to transcriptional modulation by application of a G-quadruplex-stabilizing small molecule ligand to cells. The direct structure-based approach that we have described here complements and contrasts with our recent published work that functionally links a cellular DNA damage phenotype induced by a G-quadruplex-binding ligand with G-quadruplex targets in the genome [40] . Our previous work [40] revealed targets of PDS, by ChIP-Seq analysis for the DNA damage marker, γH2AX that is recruited to large genomic regions (up to 1 Mb) on either side of the DNA damage site [42] . The antibody-based mapping of DNA G-quadruplex structures, described in the current study, has localized G-quadruplex structures at substantially finer resolution as the location of a G-quadruplex can be mapped to within a few hundred base pairs, with almost all of the peaks obtained being <2 kb in length as compared with the γH2AX peaks, which were generally greater than tens of kilobases. The examples of peaks in Fig. 2 show close overlap of the peaks to the predicted G-quadruplex regions. Furthermore, as the majority of peaks (56.6%) correspond to genomic regions with only a single G-quadruplex, the current strategy shows increased sensitivity compared with our previous study, where only large G-rich clusters comprising multiple G-quadruplexes were detected. To the best of our knowledge, our studies provide the only examples of direct G-quadruplex structure mapping in genomic DNA. It should be noted that the antibody-based mapping described here can also detect genomic regions containing clusters of G-quadruplex structures. For example, of the G-quadruplex-containing peaks isolated by hf2, 24 are predicted to fold into more than five simultaneous G-quadruplexes ( Supplementary Table S4 ). Eleven of these clusters are positioned within the sub-telomeres, regions which are known to be G-rich and contain many copies of degenerate telomeric repeats (TTAGGG). For telomeres, sequencing is not the best approach to unambiguously map these highly repetitive elements to the genome, and alternative approaches have provided evidence for the formation and functional role of G-quadruplexes at telomeres across species [43] , [44] , [45] . However, our results obtained through qPCR analysis (described above) indeed show that telomeres are enriched by at least 20-fold with the hf2 G-quadruplex structure probes. This localization of stable G-quadruplexes to telomeres and sub-telomeres underpins recent findings in human cells that these regions are enriched in recognition sites for the ATRX, a SWI/SNF family protein known to bind G-quadruplexes in vitro [46] . These results go a considerable way towards addressing a fundamental question as to whether G-quadruplex structures can form in the context of double-stranded DNA, especially given the particularly stable nature of GC-rich DNA. That double-stranded genomic DNA fragments have been isolated and enriched in this study by virtue of containing a folded G-quadruplex structure, confirms that G-quadruplexes can stably exist within genomic DNA in the presence of the complementary strand. This is in-line with previous biophysical studies that employed synthetic DNA oligonucleotides to show that G-quadruplex structures could form in the context of double-stranded DNA [47] , [48] , [49] . Clearly, the higher order organization of chromatin, the interactions with associated proteins as well as the torsional and functional status of a region of genomic DNA will have a major role in dictating where and when G-quadruplexes might form in cellular genomic DNA. We conclude that long-lived G-quadruplex structures exist and can be detected with precision in human genomic DNA. ELISA The hf2 antibody plasmid construct from Fernando et al . [11] was transformed into chemically competent BL21(DE3) E.coli cells (Bioline). Protein expression was induced using 1 mM IPTG with overnight culture at 30 °C. After centrifugation at 10,000 g for 30 min, hf2 antibody was purified from the culture supernatant using protein A-sepharose beads (Sigma-Aldrich). After washing beads with 50 mM KH 2 PO 4 , 100 mM KCl, pH 7.4, the hf2 antibody was eluted with 0.1 M tricine, pH 3.0 into 0.1 M KH 2 PO 4 pH 8.0. Biotinylated oligonucleotides (Sigma-Aldrich) for sequences known to form G-quadruplexes in vitro , and control sequences not predicted to form G-quadruplexes, were annealed in 10 mM Tris pH 7.4, 100 mM KCl by heating to 95 °C for 10 min, then cooled slowly to room temperature overnight. High Bind StreptaWell plates (Roche) were coated with 50 nM biotinylated oligonucleoties for 1 h then washed three times with ELISA buffer (50 mM K 2 HPO 4 pH 7.4 and 100 mM KCl). Wells were blocked in 3% BSA in ELISA buffer for 2 h then incubated with a serial dilution of the hf2 antibody up to 200 nM for 1 h. After three washes with ELISA buffer plus 0.1% tween, wells were incubated with 1:5,000 dilution of protein A-HRP (Life Technologies) for 1 h. After three washes with ELISA buffer plus 0.1% tween, the bound protein A-HRP was detected with the substrate TMB. The absorbance at 450 nm was measured with a plate reader (Tecan). Sequences of oligonucleotides for ELISA KIT-2 CGGGCGGGCGCGAGGGAGGGG; Htelo GGGTTAGGGTTAGGGTTAGGGTTAGGGTTAG; BCL2 GGGCGCGGGAGGAATTGGGCGGG; MYC TGAGGGTGGGTAGGGTGGGTAA. Pull-down of oligonucleotides Oligonucleotides (Sigma-Aldrich) for sequences known to form G-quadruplexes in vitro and control sequences were annealed as above. Salmon sperm DNA (Fisher Scientific) was re-suspended in 10 mM Tris pH 7.4 and sonicated with the Bioruptor UCD200 sonicator (Diagenode) for 60 min at high power with a pulse of 30 s on/30 s off, to produce fragments of ~200 bp. 100–200 pmol of hf2 was incubated with 15–50 pmol of annealed oligonucleotides with rotation for 2 h. Protein-A dynabeads (Life Technologies) were washed three times with PBS then blocked in 0.5% BSA in PBS for 2 h. Beads were added to the hf2/oligonucleotide mix and incubated rotating for 1 h. After four washes with 10 mM Tris pH 7.4, 100 mM KCl, 0.1% tween, bound oligonucleotides were eluted in 1% SDS, 0.1 M NaHCO 3 and analysed by electrophoresis in 12% TBE-urea gels. Sequences of oligonucleotides for pull-down: KIT-2 GGGCGGGCGCGAGGGAGGGG; ssDNA GCACGCGTATCTTTTTGGCGCAGGTG; dsDNA ACGAAGTTATACGCGTCGTCGAC; KIT-1+2 CGGGCGGGCGCGAGGGAGGGGAGGCGAGGAGG GGCGTGGCCGGCGCGCAGAGGGAGGGCGCTGGGAGGAGGGGC; Htelo TTAGGGTTAGGGTTAGGGTTAGGGTTAGGGTTAGG GTTAGGGTTAGGGTTAGGGTTAGGGTTAGGGTTAGGGTTAGGGTTAGGGTTAGGGTTAGGGTTAG. Cell culture and genomic DNA isolation Human breast adenocarcinoma (MCF7) cells were obtained from the European Collection of Animal Cell Cultures and grown in Dulbecco’s Modified Eagle’s Media supplemented with 10% fetal calf serum (Sigma-Aldrich) at 37 °C in 5% CO 2 . Genomic DNA was extracted from MCF7 cells using QIAamp DNA Mini Kit (Qiagen) according to the manufacturer’s protocol. The purified DNA was eluted from columns in 10 mM Tris pH 7.4. Genomic DNA was sheared by sonication as above before pull-down experiment. Pulldown of genomic DNA Fifty microliter of Protein A Dynabeads were washed three times with PBS then incubated with 2.5 μg of hf2 in 0.5% BSA and 1 mg ml −1 yeast tRNA in PBS overnight rotating at 4 °C. Beads were washed three times with 0.5% BSA then incubated with 400 μl of 300 ng μl −1 sonicated genomic DNA. Following overnight incubation rotating at 4 °C, beads were washed six times with 10 mM Tris pH 7.4, 100 mM KCl, 0.1% tween then once with 10 mM Tris pH 7.4, 100 mM KCl. Bound DNA was eluted in 50 μl of 1% SDS, 0.1 M NaHCO 3 at 30 °C for 1 h then purified with Roche PCR purification columns. Recovered DNA was assessed for enrichment of telomeric sequences by qPCR with primers for telomeric repeats and a control genomic region in a regulatory region of the oestrogen receptor gene without predicted G-quadruplex sequences. Recovered DNA was used to prepare libraries for Illumina sequencing using the TruSeq DNA library kit. Library quality was assessed using an Agilent Bioanalyzer 2100 before single end 36 base sequencing on the Illumina MiSeq, GAIIx or HiSeq 2000. Sequences of oligonucleotides for PCR: tel 1 GGTTTTTGAGGGTGAGGGTGAGGGTGAGGGTGAGGGT; tel 2 TCCCGACTATCCCTATCCCTATCCCTATCCCTATCCCTA; ESR Fw GAAACAGCCCCAAATCTCAA; ESR Rv TTGTAGCCAGCAAGCAAATG. Analysis of Illumina sequencing data Four independent pull-down and one input control libraries were analysed. Fastq files generated by the Illumina pipeline (CASAVA 1.7 and OLB 1.9.4) were aligned against the Human Reference Genome (assembly hg18, NCBI build 36.1, March 2008) using bwa [50] with default parameters. Reads not assigned to a single genomic position (that is, with MAPQ<15) were discarded. Reads overlapping regions with unusually large numbers of reads independent of the antibody used were also discarded ( http://hgdownload-test.cse.ucsc.edu/goldenPath/hg18/encodeDCC/wgEncodeMapability/wgEncodeDukeRegionsExcluded.bed6.gz ). Quality metrics for the four libraries sequence are summarized in Supplementary Table S1 . To minimize biases in the detection of enriched regions caused by unequal library sizes [51] , libraries were down-sampled to eight million reads using Picard/DownsampleSam ( http://picard.sourceforge.net/command-line-overview.shtml#DownsampleSam ). Peak-calling was performed using MACS 1.4 [17] with default settings and the input library as control. The motif discovery tool MEME [52] was used to identify common sequence motifs in the peaks. Circular dichroism Oligonucleotides (10 μM) for sequences predicted to form G-quadruplexes present in the peaks ( Supplementary Table S4 ) were annealed in 10 mM Lithium cacodylate pH 7.2, 1 mM EDTA and 100 mM KCl by heating to 95 °C for 10 min followed by slow cooling to room temperature overnight. The CD spectra were measured on a Chirascan spectropolarimeter in a quartz cuvette with a 1-mm optical path length. Three scans were obtained from 200 to 315 nm at 25 °C for each sample with a step size of 1 nm, a time per point of 1 s and a bandwidth of 0.5 nm. The scans were averaged and the spectrum obtained with a buffer only sample was subtracted with zero-correction at 315 nm. Pyridostatin treatment and qRT–PCR MCF7 cells (2 × 10 5 per well) were plated in six-well plates and cultured with 10 μM PDS or 0.1% DMSO for 24 h. Total RNA was isolated using the RNeasy mini kit (Qiagen, Crawley, UK) and 2 μg RNA used for cDNA synthesis using the Maxima reverse transcriptase (Fermentas) with random hexamers following the manufacturers’ instructions. Quantitative real-time PCR (qRT–PCR) was performed using Fast SYBR PCR mix (Applied Biosystems, UK), with a BioRad CFX96 quantitative PCR machine. Cycling conditions were 95 °C for 20 s followed by 40 cycles of 3 s at 95 °C and 30 s at 60 °C. Pyridostatin-treated and control samples were analysed in triplicate and the results analysed with the BioRad CFX software. Sequences of oligonucleotides used for qRT–PCR: ABCG1 Forward TCAGGGACCTTTCCTATTCG; ABCG1 Reverse TTCCTTTCAGGAGGGTCTTGT; ACTB1 Forward Qiagen primer set QT00193473; ACTB1 Reverse Qiagen primer set QT00193473; ACTN1 Forward GGGTTATGATATTGGCAACGA; ACTN1 Reverse TTGGGGTCCACAATGCTC; B2M Forward Qiagen primer set QT00088935; B2M Reverse Qiagen primer set QT00088935; DYSF Forward TTCGAAAGCCTCAGACTTGG; DYSF Reverse GGGACTGCCATAGAGGTTGA; ELL Forward CCGAAGTGCCATTGTCATC; ELL Reverse CCGAAACTGAACCTTCTTGC; LRP1 Forward CGCTGCATCAACACTCATGG; LRP1 Reverse AACGGTTCCTCGTCAGTCAC; PVT1 Forward AGAATCCGTGTCTGGGAGAA; PVT1 Reverse TCCCCTTAATAGTTGGCTTCC; RPLP0 Forward CCTCGTGGAAGTGACATCGT; RPLP0 Reverse CTGTCTTCCCTGGGCATCAC; STARD8 Forward GCCTCTTTTAGCCTCGTCCC; STARD8 Reverse TGGGAAGCACTTCACCTTCC; TOM1 Forward TGATGCTGGCTCTCACAGTC; TOM1 Reverse GGTCCTCACCAGCACACTCT. Accession codes: Sequencing and processed data have been submitted to the NCBI Gene Expression Omnibus under accession code GSE45241 . How to cite this article: Lam, E. Y. N. et al . G-Quadruplex structures are stable and detectable in human genomic DNA. Nat. Commun. 4:1796 doi: 10.1038/ncomms2792 (2013).